Developmental enhancers revealed by extensive DNA methylome maps of zebrafish early embryos DNA methylation undergoes dynamic changes during development and cell differentiation. Recent genome-wide studies discovered that tissue-specific differentially methylated regions (DMRs) often overlap tissue-specific distal cis -regulatory elements. However, developmental DNA methylation dynamics of the majority of the genomic CpGs outside gene promoters and CpG islands has not been extensively characterized. Here, we generate and compare comprehensive DNA methylome maps of zebrafish developing embryos. From these maps, we identify thousands of developmental stage-specific DMRs (dsDMRs) across zebrafish developmental stages. The dsDMRs contain evolutionarily conserved sequences, are associated with developmental genes and are marked with active enhancer histone posttranslational modifications. Their methylation pattern correlates much stronger than promoter methylation with expression of putative target genes. When tested in vivo using a transgenic zebrafish assay, 20 out of 20 selected candidate dsDMRs exhibit functional enhancer activities. Our data suggest that developmental enhancers are a major target of DNA methylation changes during embryogenesis. Enhancers are DNA sequences that can influence transcription of nearby genes in an orientation- and position-independent manner. Enhancers can activate transcription of their target genes from long distances [1] and play essential roles in driving spatial and temporal patterns of gene expression during development [2] . As the location of enhancers relative to their target genes is highly variable and the activity of enhancers can be restricted to a specific cell type or a specific developmental stage, the identification of enhancers has been challenging [3] . Comparative genomic studies found that non-coding sequences that are highly conserved between different species were enriched for enhancers [4] , [5] , but only a small fraction was validated as functional enhancers in transgenic mouse reporter assays [6] . Furthermore, many functional enhancers showed modest or no sequence conservation between species [7] . Chromatin immunoprecipitation followed by high-throughput sequencing (ChIP-seq) of specific epigenomic marks such as histone H3 mono-methylated lysine 4 (H3K4me1) [8] or p300 (ref. 9 ) has also been used to identify enhancers. Recent efforts in annotating genome-wide enhancers in a variety of cell types, including those of the ENCODE project, identified hundreds of thousands putative enhancers in human and mouse [10] , [11] . However, the majority of these predicted enhancers are still waiting to be tested by in vivo enhancer assays; a substantial portion of tested ones failed to be validated as active enhancers in vivo [12] . Thus, current enhancer prediction methods have both high false-negative rate (missed enhancers) and high false-positive rate (validated as non-enhancers in other assays) [13] . This implies that alternative methods to predict active and functional enhancers in a certain cell type or at a certain developing stage need to be considered, to complement and enhance the efficacy of the existing methods. DNA methylation is one of the best-studied epigenetic modifications. It plays crucial roles in diverse biological processes, including transcription, tissue-specific gene expression and normal development [14] . Methylated DNA sequences in the genome differ between different cell types and developmental stages [15] , [16] . DNA methylation is known to define and stabilize cellular identity and developmental state [17] . Until recently, many studies on DNA methylation focused on CpG-rich regions such as CpG islands (CGIs) and transcription start sites (TSSs), and only a few recent studies investigated DNA methylation on other genomic features [18] , [19] , [20] , [21] , [22] . For example, gene body methylation can be tissue specific and plays an important role in regulating intragenic promoter activity [18] . DNA methylation signatures of distal regulatory elements began to emerge from several recent studies [18] , [19] , [20] , [21] , [22] , [23] . These studies suggest that DNA methylation is important in regulating enhancers. Thus, accurate detection of differential DNA methylation status across different biological states could help identify and annotate functional enhancers in different cell types and developmental stages. Indeed, recent studies investigated the epigenetic dynamics including DNA methylation in a developmental context by differentiating human embryonic stem cells [24] , [25] . However, a thorough investigation on the relationship between DNA methylation and functional enhancers in live developing embryos is still lacking. Here we use zebrafish to study DNA methylation changes during early development and investigate the potential biological function of developmental stage-specific differentially methylated regions (dsDMRs). Zebrafish have proven an outstanding model organism to study vertebrate development [26] . DNA methylation also plays an important role in normal zebrafish development. Previous studies have shown that perturbed DNA methylation in developing zebrafish embryos resulted in critical developmental defects [27] , [28] , [29] . Very recently, DNA methylation patterns of zebrafish gametes and early embryos were determined by using whole-genome bisulfite sequencing [30] , [31] . These studies discovered global DNA methylation reprogramming differences between paternal and maternal genomes in very-early zebrafish embryos. Interestingly, one study also reported that many DMRs were located in gene bodies, especially the first introns, and were overlapping with known enhancer regions, raising the possibility that those regions might include enhancers [31] . This result encouraged the thought that DNA methylation dynamics could potentially reveal important developmental regulatory elements during zebrafish development. Here we generate comprehensive DNA methylation profiles of zebrafish developing embryos and sperm by using two complementary high-throughput sequencing technologies coupled with the state-of-art computational algorithms [18] , [22] , [23] , [32] , [33] . We identify thousands of differentially methylated DNA sequences in the zebrafish genome across different developmental stages. We find that a substantial portion of dsDMRs behave as developmental enhancers, a subset of which are successfully validated using in vivo transgenic zebrafish reporter assays. These dsDMRs strongly enrich for enhancer-associated histone modifications and for binding motifs of transcription factors (TFs) involved in important developmental processes. Reconstruction of gene regulatory networks connecting these TFs and putative target genes with nearby dsDMRs demarcates epigenetic and regulatory events associated with organogenesis and signalling pathways in developing embryos. Our results suggest that the main targets of dynamic DNA methylation reprogramming in developing zebrafish embryos are developmental enhancers, and that DNA methylation dynamics can be used to reliably discover functional enhancers. DNA methylome maps of zebrafish embryogenesis To understand how DNA methylation changes during zebrafish embryogenesis, we generated high-resolution DNA methylome maps of six developmental stages: sperm, 2.5 h post fertilization (2.5 hpf, 256 cells), 3.5 hpf (high), 4.5 hpf (dome), 6 hpf (shield) and 24 hpf ( Fig. 1a ). For each developmental stage, we constructed two sequencing libraries using complementary technologies developed recently [18] : methylation-dependent DNA immunoprecipitation followed by sequencing (MeDIP-seq) and methyl-sensitive restriction enzyme digestion followed by sequencing (MRE-seq). 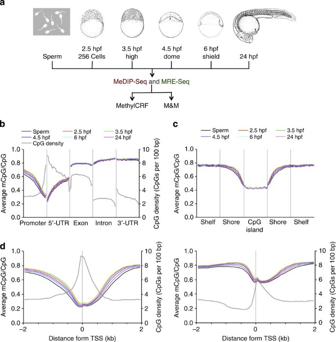Figure 1: Global features of DNA methylation across zebrafish embryogenesis. (a) A schematic representation of the study. MeDIP-seq and MRE-seq libraries were constructed from genomic DNA of six developmental stages: sperm, 2.5, 3.5, 4.5, 6 and 24 hpf. Stage-specific drawings of representative embryos are adapted from ref.26, with permission from Wiley-Liss, Inc., 1995. The two sequencing libraries for each developmental stage were further processed and analysed using recently developed algorithms, methylCRF and M&M. Both algorithms integrate MeDIP-seq and MRE-seq data. (b–d) The average DNA methylation level across different genomic features: gene-associated regions (b), CGIs and neighbouring regions (c), and high and low CpG density promoters (d). Promoter was defined as 1 kb upstream from TSS inb. CGI shore was defined as 2 kb regions flanking a CGI and CpG shelf as a 2 kb region outside a CpG shore (away from the CGI). The average CpG densities (grey lines) over the regions was also plotted inbandd. These libraries were sequenced to generate ~840 million reads in total ( Supplementary Table 1 ), which were mapped to the zebrafish genome assembly (Zv9). As shown previously, MRE-seq scores were inversely correlated with MeDIP-seq scores and the two sequencing signals covered largely non-overlapping regions ( Supplementary Figs 1 and 2 ). Figure 1: Global features of DNA methylation across zebrafish embryogenesis. ( a ) A schematic representation of the study. MeDIP-seq and MRE-seq libraries were constructed from genomic DNA of six developmental stages: sperm, 2.5, 3.5, 4.5, 6 and 24 hpf. Stage-specific drawings of representative embryos are adapted from ref. 26 , with permission from Wiley-Liss, Inc., 1995. The two sequencing libraries for each developmental stage were further processed and analysed using recently developed algorithms, methylCRF and M&M. Both algorithms integrate MeDIP-seq and MRE-seq data. ( b – d ) The average DNA methylation level across different genomic features: gene-associated regions ( b ), CGIs and neighbouring regions ( c ), and high and low CpG density promoters ( d ). Promoter was defined as 1 kb upstream from TSS in b . CGI shore was defined as 2 kb regions flanking a CGI and CpG shelf as a 2 kb region outside a CpG shore (away from the CGI). The average CpG densities (grey lines) over the regions was also plotted in b and d . Full size image Whole-genome methylation levels at single CpG resolution We used methylCRF to estimate individual methylation levels of all CpGs in the zebrafish genome by combining MRE-seq and MeDIP-seq data for each developmental stage [33] . Briefly, methylCRF uses conditional random fields to integrate MeDIP- and MRE-seq data, and predicts DNA methylation levels at single-CpG resolution. MethylCRF predictions were in high concordance with previously published predictions based on whole-genome bisulfite sequencing (MethylC-seq) [30] , [31] on the matched samples including sperm, 2.5 and 3.5 hpf embryos ( Supplementary Fig. 3a,b ). Using previously developed benchmarking metrics [33] , we determined that methylCRF and MethylC-seq were about 91% concordant within a 0.25 difference (see Methods, Supplementary Fig. 3a,b ). We found that the concordance increased with increasing MethylC-seq read depth ( Supplementary Fig. 4 ), recapitulating what was reported previously [33] . Using bisulfite-sequencing-based methods, we performed targeted validation for eight genomic regions where methylCRF and MethylC-seq predictions were discordant. The validation results agreed much better with methylCRF ( Supplementary Fig. 5 ). Taken together, these data demonstrated the high quality of our DNA methylome maps. To characterize the DNA methylation levels across different genic features, we plotted methylation levels across gene-associated regions including promoters, exons, introns, and 5′- and 3′-untranslated regions (UTRs) ( Fig. 1b ). Overall, the average genic DNA methylation levels of each developmental stage were almost identical. We observed a negative correlation in the methylation level and the proximity to the TSS. The DNA methylation level increased in the 5′-UTR and stayed high in exons, introns and the 3′-UTR, which resembled the DNA methylation pattern over genic regions in the human embryonic stem cells [34] . We also investigated the DNA methylation levels across CGIs, and CGI shores and shelves. CGIs were largely unmethylated and methylation levels increased with increasing distance from CGIs ( Fig. 1c ). Predicted DNA methylation levels were also plotted as an average profile throughout the protein-coding genes. The low DNA methylation around the TSS was observed again and the transcription termination sites had slightly higher DNA methylation levels ( Supplementary Fig. 6a ). The DNA methylation levels throughout long non-coding RNA (lncRNA) genes looked very similar to those of protein-coding genes ( Supplementary Fig. 6b ). The DNA methylation levels across different genic and genomic features shown above were further confirmed using the recently published zebrafish MethylC-seq data sets ( Supplementary Fig. 7 ). The low DNA methylation level around the TSS was correlated with high CpG density around the TSS ( Fig. 1b ). We further investigated the relationship between the DNA methylation level and the CpG density of the promoters. We divided all protein-coding gene promoters into two categories, high CpG promoters (HCPs) and low CpG promoters (LCPs) ( Supplementary Fig. 8a ), and found that LCPs were more methylated than HCPs on average ( Fig. 1d and Supplementary Fig. 8b ). This confirms that the CpG density of the promoters is negatively correlated with the DNA methylation level in mammals [35] and zebrafish [30] , [31] . Taken together, these results suggested that the global characteristic DNA methylation patterns over genic regions in zebrafish were established as early as 2.5 hpf and remained stable through early embryo development, and that the patterns were similar to those of other vertebrate animals including mouse and human. Identification of DMRs We next asked whether there are regulated local DNA methylation changes across different developmental stages. We applied to our data a recently invented integrative statistical algorithm M&M [23] . Briefly, M&M integrates MeDIP-seq and MRE-seq by dynamically scaling, normalizing and combining two data sets, and identifies DMRs between two samples. This allowed us to identify a total of 8,225 DMRs between different developmental stages (see Methods, Fig. 2a , Supplementary Fig. 9a,b and Supplementary Data 1 ). It is noteworthy that the most dramatic differences were identified between 6 and 24 hpf embryos, where the majority of over a thousand DMRs showed decreasing DNA methylation level from 6 to 24 hpf embryos, suggesting that locus-specific demethylation process could be an important feature of early cell specification and differentiation. 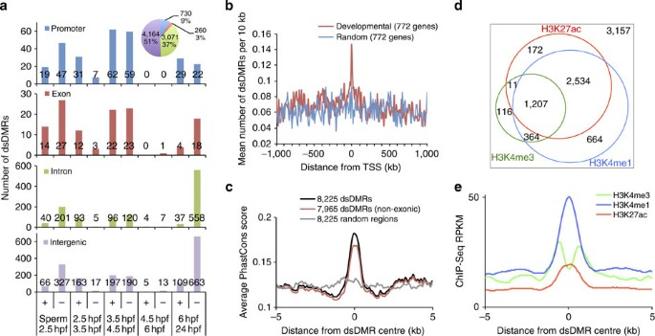Figure 2: Identification of the dsDMRs. (a) The number of dsDMRs identified between neighbouring developmental stages as indicated onxaxis. Plus sign (+) indicates dsDMRs with increasing DNA methylation levels with respect to step-wise developmental stages and minus sign (−) indicates dsDMRs with decreasing DNA methylation. The genomic locations of dsDMRs were indicated by different colours. Pie chart: the genomic locations of all DMRs identified in pair-wise comparisons. (b) The distribution of dsDMRs around genes related to embryo development (red) or around random genes (blue). (c) Sequence conservation of dsDMRs. Vertebrate PhastCons scores of the dsDMRs and their flanking 10 kb regions were averaged and plotted. (d) A weighted Venn diagram of the number of dsDMRs overlapping with histone modification peaks from any developmental stages. (e) Histone modification signature of dsDMRs. Average histone modification ChIP-seq RPKM values from 24 hpf embryos were plotted over 10 kb regions centred on dsDMRs. Figure 2: Identification of the dsDMRs. ( a ) The number of dsDMRs identified between neighbouring developmental stages as indicated on x axis. Plus sign (+) indicates dsDMRs with increasing DNA methylation levels with respect to step-wise developmental stages and minus sign (−) indicates dsDMRs with decreasing DNA methylation. The genomic locations of dsDMRs were indicated by different colours. Pie chart: the genomic locations of all DMRs identified in pair-wise comparisons. ( b ) The distribution of dsDMRs around genes related to embryo development (red) or around random genes (blue). ( c ) Sequence conservation of dsDMRs. Vertebrate PhastCons scores of the dsDMRs and their flanking 10 kb regions were averaged and plotted. ( d ) A weighted Venn diagram of the number of dsDMRs overlapping with histone modification peaks from any developmental stages. ( e ) Histone modification signature of dsDMRs. Average histone modification ChIP-seq RPKM values from 24 hpf embryos were plotted over 10 kb regions centred on dsDMRs. Full size image We then examined the enrichment of differentially methylated individual CpGs with respect to either hypermethylated or hypomethylated DMRs. Differences in methylation levels of individual CpGs showed clear separation between hypermethylated DMRs and hypomethylated DMRs ( Supplementary Fig. 9c ), confirming that our DMR set was highly specific. We thus termed these DMRs zebrafish dsDMRs. Genomic distribution of dsDMRs was highly non-random. Approximately 10% of dsDMRs were located in the gene promoter regions, whereas the remaining dsDMRs were either in intergenic or intronic regions ( Fig. 2a and Supplementary Fig. 9b ). Most dsDMRs were located 10–50 kb away from its closest TSS, but the number of dsDMRs located <1 kb from TSS was greater than expected ( Supplementary Fig. 10a ). This suggests that the promoters were enriched as a main target of DNA methylation changes during embryogenesis; however, the majority of DNA methylation changes occurred distal to gene promoters. To investigate the relationship between dsDMRs and developmental processes, we asked whether the dsDMRs were more enriched near a collection of 772 genes that were annotated as important for embryonic development (Methods). Strikingly, the distribution of dsDMRs was more significantly enriched near developmental genes than random expectation ( Fig. 2b , Kolmogorov–Smirnov test, P -value<1 × 10 −14 ). Similarly, when we compared the number of dsDMRs located within 50 kb from TSS of the developmental genes, we found that developmental genes had significantly higher number of dsDMRs than randomly chosen genes ( Supplementary Fig. 10b ). This suggests that the dsDMRs might have functions related to developmental processes. To evaluate the functional potential of the dsDMRs, we asked whether their sequences were evolutionarily conserved by examining their PhastCons scores [36] based on the eight-way vertebrate genome alignment with zebrafish from the UCSC Genome Browser [37] . A significant proportion of dsDMRs (1,546 out of 8,225) contained sequences that were evolutionarily conserved across vertebrates (hypergeometric test, P -value=6.1 × 10 −41 ). Average conservation scores of all dsDMRs were higher than their neighbouring regions ( Fig. 2c ). This trend remained after we excluded DMRs that overlapped exonic sequences ( Fig. 2c ), suggesting many dsDMRs were contributed by conserved non-coding sequences. We hypothesized that dsDMRs may encode important regulatory elements for developmental functions. We thus examined histone posttranslational modifications on dsDMRs using publicly available ChIP-seq data on four zebrafish embryonic developing stages: dome (4.5 hpf), 80% epiboly (8.5 hpf), 24 and 48 hpf [38] . More than half of the dsDMRs (4,952/8,225) overlapped with at least one enhancer-associated histone ChIP-seq peak—H3K4me1 or histone H3-acetylated lysine 27 (H3K27ac)—from at least one of the four developmental stages (hypergeometric test, P -value=4.7 × 10 −1478 ; Fig. 2d and Supplementary Fig. 10c ). Average ChIP-seq score over 10 kb regions around the DMRs identified strong peaks of H3K4me1 and H3K27ac centred on the DMRs ( Fig. 2e and Supplementary Fig. 10d,e ). This data revealed that dsDMRs were strongly associated with enhancer chromatin marks. Taken together, the genomic distribution, sequence conservation and histone modification pattern of the dsDMRs we discovered suggest that they may be regulatory elements playing important roles in developmental processes. Most dsDMRs are putative developmental enhancers Across all developmental stage step-wise comparisons, the comparison between 6 and 24 hpf embryos yielded a relatively large number of dsDMRs (a total of 1,440) and, interestingly, majority (1,261, or 88%) of them exhibited hypomethylation in 24 hpf embryos ( Fig. 2a ). As many important developmental processes including cell specification occur during this time [26] , we hypothesized that these hypomethylated dsDMRs may represent distal enhancers that were dynamic during development [20] . Consistent with this hypothesis, we found that ~70% of these dsDMRs (880 out of 1,261) directly overlapped with putative distal regulatory elements (PDREs) that were identified using enhancer histone marks [38] (hypergeometric test, P -value=1.9 × 10 −790 ). Furthermore, this group of dsDMRs had the highest percentage of dsDMRs with conserved sequences (30%, 378 out of 1,261; hypergeometric test, P -value=6.1 × 10 −52 ). The average conservation score over the 10-kb regions surrounding dsDMRs revealed strong enrichment of conserved elements over the dsDMRs ( Fig. 3a ). When compared with the conservation profile of the PDREs identified in 24 hpf, the average PhastCons scores of the dsDMRs were even higher ( Fig. 3a ). 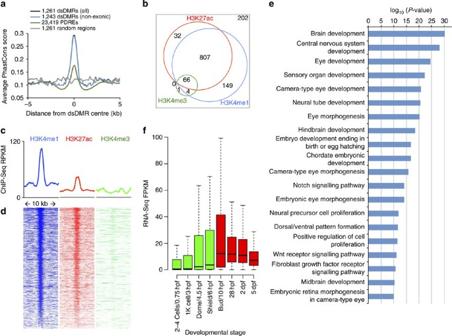Figure 3: Most dsDMRs with decreasing DNA methylation level between 6 and 24 hpf are developmental enhancers. (a) Averaged vertebrate PhastCons scores of 10 kb regions centred on dsDMRs were plotted. (b) A weighted Venn diagram of dsDMRs overlapping with different histone modification peaks from 24 hpf embryo. (c) Histone modification signature of dsDMRs. Average ChIP-seq RPKM values from 24 hpf embryos were plotted over 10 kb regions centred on the dsDMRs. (d) Heat maps of ChIP-seq signal over 10 kb regions centred on individual dsDMRs. (e) Enriched GO terms and their binomialP-values from analysing dsDMRs using GREAT42. The top 20 GO terms were displayed here and the full list of GO terms enriched was inSupplementary Fig. 11a. (f) Expression profiles of genes associated with dsDMRs from GO enrichment analysis across different developmental stages. Figure 3: Most dsDMRs with decreasing DNA methylation level between 6 and 24 hpf are developmental enhancers. ( a ) Averaged vertebrate PhastCons scores of 10 kb regions centred on dsDMRs were plotted. ( b ) A weighted Venn diagram of dsDMRs overlapping with different histone modification peaks from 24 hpf embryo. ( c ) Histone modification signature of dsDMRs. Average ChIP-seq RPKM values from 24 hpf embryos were plotted over 10 kb regions centred on the dsDMRs. ( d ) Heat maps of ChIP-seq signal over 10 kb regions centred on individual dsDMRs. ( e ) Enriched GO terms and their binomial P -values from analysing dsDMRs using GREAT [42] . The top 20 GO terms were displayed here and the full list of GO terms enriched was in Supplementary Fig. 11a . ( f ) Expression profiles of genes associated with dsDMRs from GO enrichment analysis across different developmental stages. Full size image The profiles of histone modification marks suggested that this set of dsDMRs strongly enriched for enhancer elements, much more than for promoters. Seventy eight per cent of these dsDMRs (988 out of 1,261) overlapped with either or both of the two enhancer-associated marks H3K4me1 or H3K27ac peaks in the absence of the promoter-associated mark H3K4me3 peaks (hypergeometric test, P -value=2.5 × 10 −843 ), while a smaller but still significant portion of dsDMRs overlapped with H3K4me3 peaks (hypergeometric test, P -value=9.6 × 10 −9 ; Fig. 3b ). Averaged ChIP-seq signals for the 10-kb region around these dsDMRs showed strong enrichment of H3K4me1 and H3K27ac ( Fig. 3c ), and individual dsDMRs each displayed strong enhancer-associated signal ( Fig. 3d ). To investigate whether the genes nearby these dsDMRs were enriched for any functional annotation, we performed Gene Ontology (GO) enrichment analysis on these dsDMRs by using the tool GREAT [39] . This analysis revealed that genes associated with these dsDMRs strongly enriched for many biological functions involving brain and eye development, for instance, ‘brain development’ and ‘central nervous system development’ ( Fig. 3e , Supplementary Fig. 11a,b and Supplementary Table 2 for the complete list). In addition, fibroblast growth factor receptor (FGFR), Notch and Wnt receptor signalling pathways were also enriched ( Fig. 3e and Supplementary Fig. 11a,b ). To investigate whether the genes identified from GREAT analysis might be direct targets of dsDMRs, we asked whether the expression of these genes correlated with the methylation status of the dsDMRs, by examining publically available expression profiles of developing zebrafish embryos [40] . The genes associated with these dsDMRs showed increased expression levels in 10 (bud) or 28 hpf when compared with the levels in 6 hpf (shield; Fig. 3f and Supplementary Fig. 12 ). In particular, 72 genes had no or very little RNA expression (fragments per kilo base of exon per million mapped reads (FPKM) <1) in shield stage and were activated (FPKM >1) in the later stages. Thus, the expression dynamics of genes associated with this DMR set was consistent with the hypothesis that these dsDMRs were enhancers for regulating expression of their nearby genes. Gene regulatory network derived from DNA methylome maps Given the regulatory potential of dsDMRs, we hypothesized that these dsDMR enhancers coordinate many developmental processes by connecting upstream TFs to their downstream target genes. To test this, we first identified the TF-binding motifs enriched in these dsDMRs. We found that dsDMRs were highly enriched for binding motifs of many important developmental TFs, including Sox family and nuclear receptor family proteins ( Fig. 4a and Supplementary Fig. 13 ). Zebrafish genes coding these TFs were also enriched for developmental processes such as ‘sensory organ development’ and ‘embryonic morphogenesis’ ( Supplementary Figs 14 and 15a and Methods). Thus, analysis of dsDMRs predicted many regulatory relationships among genes associated with development. We then asked whether these upstream TFs and downstream genes are known to be associated by querying databases of known TF target genes (Methods). Indeed, we found a large number of connections among the TFs and genes (2,964 edges with 233 nodes; Student’s t -test, P -value=1.65 × 10 −5 ; Supplementary Fig. 15b ), suggesting a highly connected, non-random network among the TFs and genes identified from dsDMR analysis. 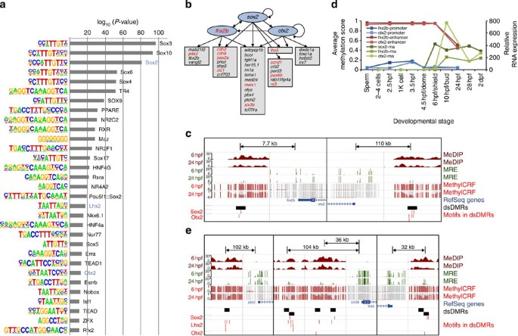Figure 4: Gene regulatory network derived by dsDMRs. (a) Enriched TF-binding motifs in dsDMRs and their hypergeometricP-values from HOMER62. On the left, sequence logo of each motif was displayed. The three motifs used in eye development regulatory network construction were indicated by blue coloured text. The motifs withP-values <10−10were displayed here and the full list of enriched motifs was inSupplementary Fig. 13. (b) The putative gene regulatory network of the eye development derived from dsDMR analysis. The blue ovals were TFs, whose motifs were enriched in dsDMRs. The genes in the grey boxes were the target genes identified in GREAT analysis. Arrows indicates that the TFs had their binding motifs in neighbouring dsDMRs of the target genes. The genes coloured in red were knownsox2target genes identified from ChEA68. (c) The gene set view of four genomic regions (chr8:3242750-3245750, chr8:3250489-3253489, chr17:44294595-44297595 and chr17:44405250-44408250) from the Epigenome browser69,70. The left panel displayed the regions aroundlhx2bpromoter and its nearby dsDMR enhancer (indicated by the black box). The right panel displayed the regions aroundotx2promoter and its nearby dsDMR enhancer. Both dsDMRs had Sox2- and Otx2-binding motifs (red ticks), suggesting thatsox2could be an upstream regulator of these two TFs. (d) The methylation profiles of thelhx2bandotx2promoters and their neighbouring dsDMR enhancers (blue and red lines, leftyaxis) and the expression profile of the two genes (green lines, rightyaxis). Each gene expression level was normalized to the expression level of 1K-cell stage. (e) The gene set view of seven genomic regions (chr13:6556250-6559250, chr13:6658232-6661232, chr13:29912750-29915750, chr13:29935250-29940750, chr13:29993060-29996060, chr13:30062750-30065750 and chr13:30077750-30080750) from the Epigenome browser69,70. The displays ofpitx3(left),six3b(middle) andlhx5(right) promoters and their nearby dsDMR enhancers were as inc. Figure 4: Gene regulatory network derived by dsDMRs. ( a ) Enriched TF-binding motifs in dsDMRs and their hypergeometric P -values from HOMER [62] . On the left, sequence logo of each motif was displayed. The three motifs used in eye development regulatory network construction were indicated by blue coloured text. The motifs with P -values <10 −10 were displayed here and the full list of enriched motifs was in Supplementary Fig. 13 . ( b ) The putative gene regulatory network of the eye development derived from dsDMR analysis. The blue ovals were TFs, whose motifs were enriched in dsDMRs. The genes in the grey boxes were the target genes identified in GREAT analysis. Arrows indicates that the TFs had their binding motifs in neighbouring dsDMRs of the target genes. The genes coloured in red were known sox2 target genes identified from ChEA [68] . ( c ) The gene set view of four genomic regions (chr8:3242750-3245750, chr8:3250489-3253489, chr17:44294595-44297595 and chr17:44405250-44408250) from the Epigenome browser [69] , [70] . The left panel displayed the regions around lhx2b promoter and its nearby dsDMR enhancer (indicated by the black box). The right panel displayed the regions around otx2 promoter and its nearby dsDMR enhancer. Both dsDMRs had Sox2- and Otx2-binding motifs (red ticks), suggesting that sox2 could be an upstream regulator of these two TFs. ( d ) The methylation profiles of the lhx2b and otx2 promoters and their neighbouring dsDMR enhancers (blue and red lines, left y axis) and the expression profile of the two genes (green lines, right y axis). Each gene expression level was normalized to the expression level of 1K-cell stage. ( e ) The gene set view of seven genomic regions (chr13:6556250-6559250, chr13:6658232-6661232, chr13:29912750-29915750, chr13:29935250-29940750, chr13:29993060-29996060, chr13:30062750-30065750 and chr13:30077750-30080750) from the Epigenome browser [69] , [70] . The displays of pitx3 (left), six3b (middle) and lhx5 (right) promoters and their nearby dsDMR enhancers were as in c . Full size image Interestingly, we found that several GO terms (either the same or closely related terms) were enriched both in the TFs predicted to bind dsDMRs and in the genes predicted to be the targets of dsDMRs ( Fig. 3e and Supplementary Figs 11a,14 and 15a ). This result further supports that our method could link TFs to their targets in the context of a specific biological process. For example, we found that the GO terms ‘eye development’ and ‘eye morphogenesis’ were enriched in both TFs that were upstream of dsDMRs and in putative target genes that were downstream of dsDMRs. This result is consistent with the hypothesis that TFs involved in eye development bind to dsDMRs, to regulate their downstream target genes. To further test whether dsDMRs coordinate the expressions of genes associated with the eye development, we sought to construct a gene regulatory network by directly linking TFs and their target genes (Methods). We identified a total of 75 links between 3 TFs and their 35 target genes, and constructed a putative gene regulatory network of eye development using these links ( Fig. 4b ). Interestingly, the majority of dsDMRs containing TF-binding motifs were located far away from the TSS of target genes, highlighting the importance of these dynamically regulated distal enhancers in mediating eye development ( Supplementary Fig. 16a ). In this regulatory network, the TFs sox2 , lhx2b and otx2 coordinated the expression of genes involved in eye development ( Fig. 4b ). All three TFs also had Sox2 motifs in their neighbouring dsDMRs ( Fig. 4c ), suggesting that sox2 is the upstream regulator of this network. Further supporting this hypothesis, we found that transcription of sox2 started in 6 hpf (shield), which was followed by demethylation of dsDMRs that contained sox2 -binding motif ( Fig. 4d ). The expression levels of lhx2b and otx2 were inversely correlated with the methylation levels of their neighbouring dsDMRs, but were not correlated with the methylation levels of their own promoters ( Fig. 4d ), underscoring the regulatory potential of these dsDMRs. All downstream target genes had one or more binding motifs of the TFs sox2 , lhx2b and otx2 in their neighbouring dsDMRs ( Fig. 4b,e ) and the expression dynamics of these genes were correlated with methylation changes of neighbouring dsDMRs ( Fig. 3f and Supplementary Fig. 16b ). This data is consistent with the hypothesis that these genes are downstream target genes of the three TFs. Our analysis not only provided regulatory connections among genes known to involve in a developmental process, but also brought novel genes into the network. For example, sema6a was not curated to share a GO term with eye developmental genes. However, we predicted that sema6a is an eye developmental gene, because a dsDMR with binding motifs of the three TFs, Sox2, Lhx2 and Otx2, was associated with sema6a gene ( Supplementary Fig. 17a ). Indeed, sema6a is a transmembrane signalling protein, which is important for mammalian retinal circuits assembly [41] and is also required for zebrafish eye cohesion [42] . In addition, the expression levels of sema6a were inversely correlated with the methylation levels of their neighbouring dsDMRs ( Supplementary Fig. 17b ). Thus, we were able to put sema6a in the eye development regulatory network. Similarly, we added cdon and ascl1b to the eye development network ( Supplementary Fig. 17a,c,d ). These two genes were not annotated by GO as eye developmental genes. However, cdon defines the correct proximo-distal patterning of the eye [43] and Ascl1 is required for specification of the mammalian retina progenitors [44] . Thus, our dsDMR-based analysis was able to construct a high-quality gene regulatory network for eye development. In addition to eye development, we were also able to construct gene regulatory networks for other developmental processes. For example, we identified 33 links between 3 TFs and 12 target genes associated with central nervous system neuron differentiation and built a putative regulatory network ( Supplementary Fig. 18 ). These findings highlight that the gene regulatory networks can be derived by analysing epigenomic changes across developmental courses. In vivo validation of dsDMRs as putative enhancer elements We next tested whether the dsDMRs could function as developmental enhancers in live zebrafish. To this end, we chose 20 dsDMRs that were associated with 8 developmental genes. For this assay, we chose dsDMRs far from the promoters (from at least 3 kb away to more than 200 kb away, Table 1 and Supplementary Tables 3–5 ). We also included four dsDMRs that did not overlap with any conserved element in this test and five dsDMRs that did not have overlapping enhancer histone peaks ( Supplementary Table 4 ). We cloned these dsDMR sequences into a minimal promoter-driven green fluorescent protein (GFP) reporter cassette [45] , [46] and injected zebrafish embryos with the reporter vector along with Tol2 transposase messenger RNA. In addition, as negative controls we also cloned 20 regions selected from within the vicinity of the tested dsDMRs but did not exhibit DNA methylation change ( Supplementary Table 3 ). These non-dsDMR negative controls included regions that overlapped with conserved element or enhancer histone peaks ( Supplementary Table 4 ). Each group of G0 embryos injected with a specific putative enhancer reporter construct expressed GFP in a specific pattern, suggesting that the transgene integration occurred early and often in embryonic development [47] . In contrast, G0 embryos injected with the negative controls showed, if any, inconsistent patterns of GFP expression ( Supplementary Fig. 19 ). We were able to establish founder G1 transgenic fish expressing GFP for all 20 putative enhancer reporter constructs. Overall, the GFP expression pattern driven by each dsDMR enhancer recapitulated the expression pattern of its adjacent gene ( Fig. 5 , Supplementary Fig. 20 and Supplementary Table 6 ). Interestingly, all of the four dsDMRs without conserved sequences ( fgfr2-e1 , fgfr2-e2 , fgfr2-e4 and sox2-e2 ) showed in vivo enhancer activities ( Fig. 5e and Supplementary Fig. 20i ). We note that we paired each dsDMR enhancer with its closest putative target gene but the enhancer may have different or additional target genes. This explains the few, if any, differences between GFP expression patterns driven by dsDMR enhancers and those of the neighbouring genes. Table 1 The dsDMR enhancers validated in vivo . 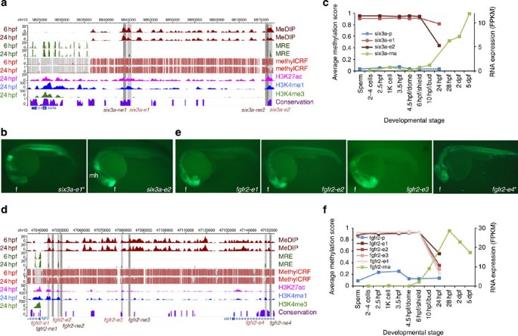Figure 5:In-vivovalidation of dsDMR enhancers. (a) Epigenome Browser69,70view of thesix3agene, neighbouring dsDMR enhancers (six3a-e1andsix3a-e2, grey boxes) and cloned region for a negative control (six3a-ne1andsix3a-ne2, dark grey boxes). (b) GFP expression driven by the dsDMR enhancers of thesix3agene. Scale bar, 200 μm. (c) The methylation profiles of thesix3apromoter and neighbouring dsDMR enhancers (blue and red lines, leftyaxis) and the expression profile of thesix3agene (green line, rightyaxis). (d) Epigenome Browser view of thefgfr2gene, neighbouring dsDMR enhancers (fgfr2-e1,fgfr2-e2,fgfr2-e3andfgfr2-e4, grey boxes) and cloned regions for negative controls (fgfr2-ne1,fgfr2-ne2,fgfr2-ne3andfgfr2-ne4, dark grey boxes). (e) GFP expression driven by the dsDMR enhancers of thefgfr2gene. (f) The methylation profiles of thefgfr2promoter and neighbouring dsDMR enhancers (blue and red lines, leftyaxis) and the expression profile of thefgfr2gene (green line, rightyaxis). *Only one G1 transgenic line was established. Forebrain (f); midbrain–hindbrain boundary (mh). Full size table Figure 5: In-vivo validation of dsDMR enhancers. ( a ) Epigenome Browser [69] , [70] view of the six3a gene, neighbouring dsDMR enhancers ( six3a-e1 and six3a-e2 , grey boxes) and cloned region for a negative control ( six3a-ne1 and six3a-ne2 , dark grey boxes). ( b ) GFP expression driven by the dsDMR enhancers of the six3a gene. Scale bar, 200 μm. ( c ) The methylation profiles of the six3a promoter and neighbouring dsDMR enhancers (blue and red lines, left y axis) and the expression profile of the six3a gene (green line, right y axis). ( d ) Epigenome Browser view of the fgfr2 gene, neighbouring dsDMR enhancers ( fgfr2-e1 , fgfr2-e2 , fgfr2-e3 and fgfr2-e4 , grey boxes) and cloned regions for negative controls ( fgfr2-ne1 , fgfr2-ne2 , fgfr2-ne3 and fgfr2-ne4 , dark grey boxes). ( e ) GFP expression driven by the dsDMR enhancers of the fgfr2 gene. ( f ) The methylation profiles of the fgfr2 promoter and neighbouring dsDMR enhancers (blue and red lines, left y axis) and the expression profile of the fgfr2 gene (green line, right y axis). *Only one G1 transgenic line was established. Forebrain (f); midbrain–hindbrain boundary (mh). Full size image We further illustrate our results with the following examples. The six3a and six3b genes play essential roles in the patterning of forebrain and eye development in many species, including zebrafish [48] . The six3a gene is expressed in the forebrain, midbrain–hindbrain boundary, anterior neural tube and medial longitudinal fasciculus, and the six3b gene is expressed in the eyes, optic stalk, optic cup, forebrain, telencephalon and diencephalon at 24 hpf ( Supplementary Table 6 ). We tested two dsDMRs upstream of the six3a gene and two dsDMRs upstream of six3b gene. Each of these dsDMRs displayed enhancer activity in similar tissue-specific patterns at 24 hpf, driving expression patterns similar to that of the endogenous gene. However, each dsDMR enhancer drove distinct subset of the endogenous expression pattern, resulting in distinct GFP expression patterns ( Fig. 5a,b and Supplementary Fig. 20a,b ). RNA expression analysis [40] confirmed that these genes were mostly silenced from 2- to 4-cell stage until shield (~6 hpf, six3b ) or bud (~10 hpf, six3a ) and were activated between shield and 28 hpf ( Fig. 5c and Supplementary Fig. 20c ). Importantly, the promoter regions of both genes remained unmethylated across developmental stages; only the dsDMR enhancers exhibited dynamic DNA methylation changes, which correlated well with gene expression ( Fig. 5c and Supplementary Fig. 20a ). Thus, DNA methylation of these enhancers could potentially regulate the spatial expression of six3 genes. The three dsDMRs upstream of the fgfr2 gene and one dsDMR upstream of the fgf3 gene also displayed enhancer activities in transgenic G1 fish ( Fig. 5d–f and Supplementary Fig. 20d,e ). FGFR signalling pathways play important roles in diverse developmental processes, including cell growth, differentiation, patterning or cell migration in vertebrates [49] . The fgfr2 gene is expressed in the forebrain, hindbrain, diencephalon and solid lens vesicle, and the fgf3 gene is expressed in the forebrain, midbrain and midbrain–hindbrain boundary ( Supplementary Table 6 ). The same overall expression patterns were observed in the G1 transgenic fish, but each enhancer drove only a subset of the full expression pattern ( Fig. 5e and Supplementary Fig. 20e ). Overall, expression patterns driven by the tested enhancers were similar to the expression patterns of their nearby putative target genes ( Supplementary Fig. 20 and Supplementary Table 6 ). Taken together, these data demonstrated that the dsDMR enhancers identified in this study were functional in a specific developmental stage; they were probably tissue-specific enhancers for spatial regulation of expression of important developmental genes. Dynamic changes of DNA methylation play a key role in normal development and cell differentiation by defining cell-type identities. DNA methylation has been extensively studied across developmental times, but until recently, most work has been focused on gene promoters and CpG islands and little is known about DNA methylation changes in intergenic regions. In this study, we comprehensively defined the genome-wide dynamics of DNA methylation in developing zebrafish embryos. We identified thousands of specific genomic regions (dsDMRs) whose methylation status underwent orchestrated changes across developmental stages. Surprisingly, the majority of dsDMRs were located outside gene promoters, CpG islands and island shores. Although the primary signal we relied on was DNA methylation, dsDMRs we identified also strongly enriched for sequence conservation, enhancer histone marks and association with developmental TFs and other developmental genes. Our transgenic zebrafish reporter assay provided strong evidence that these dsDMRs were functional developmental enhancers. Our study established that DNA methylation of enhancer elements is a major regulatory mechanism during vertebrate embryo development. Many dsDMRs we identified were from the later developmental stages, such as 24 hpf embryos. As the embryos at this stage are not homogeneous and have diverse cell types and tissues, it is possible that dsDMRs we reported here reflect specificity of the dominant cell types or development of major structures such as neurons and the eye. As technologies to isolate individual cell types continue to advance, it would be interesting and important to revisit DNA methylation dynamics of developmental enhancers in a cell type-specific manner. The DNA methylome maps of whole developing embryos, together with previously published histone modification ChIP-seq [41] and RNA-seq [43] profiling of the whole embryos, will provide an invaluable resource and reference for current and future investigations. Using MethylC-seq, Potok et al. [31] identified 9,013 DMRs in the earlier developmental stages, with many representing the difference between gametes (that is, sperm and egg). Interestingly, these early developmental DMRs had only 431 overlaps with dsDMRs identified by our study. Majority of the early DMRs reported by Potok et al. [31] did not undergo DNA methylation changes during later developmental stages profiled in our study ( Supplementary Fig. 21a ). The 431 overlapping regions ( Supplementary Fig. 21b ) showed DNA methylation changes mainly in 24 hpf embryos and the patterns were very similar to those between sperm and egg or between embryos and muscle ( Supplementary Fig. 21c ). Thus, the overlapping DMRs would mark regions associated with germline specification (hypermethylation in 24 hpf) or regions associated with muscle development (hypomethylation in 24 hpf). We conclude that our dsDMRs are overall distinct regions from the earlier-stage DMRs with a few expected overlaps. It is also noteworthy that zebrafish might use different mechanisms of DNA methylation reprogramming in early versus late embryonic developing stages. It was reported that 5-hydroxymethylcytosine (5hmC), the intermediate catalysed by the tet enzymes in DNA demethylation process, is not involved in the DNA reprogramming in earlier embryos [30] , [31] . The low expression levels of the three zebrafish tet genes across these developmental stages further supported this idea ( Supplementary Fig. 22a ). However, tet expression levels increased sharply between 6 (shield) and 28 hpf, and were inversely correlated with the methylation levels of dsDMRs analysed in our study ( Supplementary Fig. 22a,b ). This raises the possibility that 5hmC mediates active DNA demethylation in later embryos, but not in earlier embryos. Further investigation will be required to elucidate the mechanisms of DNA methylation dynamics in zebrafish embryogenesis. Previous studies have also identified several thousand putative developmental enhancers in zebrafish, named PDREs, by using three histone modifications: H3K4me1, H3K4me3 and H3K27ac [38] . The dsDMR enhancers we reported here had a significant overlap with the PDREs, but the two sets were not identical ( Supplementary Fig. 23 ). Five of 18 PDREs previously tested in stable transgenic assays were identified as dsDMRs in our study (regions 1, 2, 10, 11 and 12 in ref. 38 ) and 4 of them were validated as functional enhancers in 24 hpf embryos. We tested the in vivo enhancer activity of 20 of our dsDMRs associated with 8 important developmental genes. We were able to establish stable transgenic lines for 20 dsDMRs, and all 20 exhibited tissue-specific enhancer activities. Thus, our validation rate was higher than what was reported in the previous study (67%) [38] . Although the number of validated enhancers remained small due to the low throughput nature of the transgenic experiment, our results suggest that DNA methylation dynamics can be a robust indicator of functional enhancers, possibly more specific than histone modification alone. Therefore, integrating DNA methylation, histone modification and sequence conservation could be a more effective strategy for defining cell-type-specific or developmental stage-specific enhancers. Our study joins several recent works in supporting this idea. For example, by investigating intergenic hypomethylated regions in various human cell types, Schlesinger et al. [50] suggested that de novo DNA demethylation defines distal regulatory elements. Hon et al. [51] pointed out that identifying tissue-specific DMRs can be an alternative strategy for finding putative regulatory elements. The study showed that the enhancer-predicting resolution of tissue-specific DMRs were comparable to that of p300-binding sites and were much higher than that of using histone modifications. However, detecting putative enhancers based on differential DNA methylation requires CpGs in the primary sequences. The efficacy of such methods for CpG-poor enhancers remains to be examined. Sequence conservation has long been used to predict functional elements including enhancers. For example, Pennacchio et al. [6] tested in vivo enhancer activities of human conserved non-coding sequences in a transgenic mouse enhancer assay and found that 45% of tested sequences exhibit tissue-specific enhancer activities. Similar results were reported elsewhere [52] , [53] . However, it has been difficult to evaluate how many functional elements were missed by this type of approaches. Our results suggested that a large fraction of dsDMRs are not evolutionarily conserved at primary sequence level. However, they may still be functional developmental enhancers; we validated four such examples in this study ( Supplementary Table 4 ). DNA methylation at gene promoters has long been known to silence genes by blocking transcription [54] . In contrast, the relationship between DNA methylation at distal enhancers and gene expression remains less explored. In this study, we demonstrated that there is a positive correlation between DNA demethylation in enhancers and expression level of nearby genes ( Fig. 3f ). However, the impact of enhancer DNA methylation on gene expression is much more complex than a simple ‘on and off’ switch. Instead, enhancer DNA methylation might act more similar to a ‘dial’ that can fine-tune the expression of genes in a specific cell type and developmental time. For example, fgf3 gene expression levels across developmental courses did not correlate well with the DNA methylation status of the predicted enhancer ( Supplementary Fig. 20d,f ). This might be due to the fact that gene expression is regulated in a temporal- and spatial-specific manner, but the existing RNA expression data were from the whole embryos. It is also possible that we did not identify the bona fide target genes for some enhancers, especially when some enhancers function independently of orientation and at great distances from their target genes. In addition, some enhancers validated in our study may have additional target genes. Although DNA methylation has long been investigated in the context of gene promoters and CpG islands, only recently have studies emerged on DNA methylation signatures of enhancers. DNA hypomethylation has been observed in PDREs and tissue-specific enhancers are hypomethylated in a tissue-specific manner [20] , [22] , [23] , [24] , [25] , [55] , [56] . In line with these studies, our study provided the first evidence that functional enhancers undergo demethylation during embryogenesis. Importantly, to our knowledge, this is the first time the principle of enhancer–DNA methylation relationship is revealed in live developing embryos. These results led us to further ask the relationship between DNA methylation and enhancer activity. A recent study has shown that demethylation of distal enhancers induced by binding of glucocorticoid receptors leads to activation of the enhancer function [21] . In addition, 5hmC and the TET proteins are frequently found at distal enhancers, suggesting that demethylation of these elements is closely related to their function [56] , [57] . However, a recent study also suggested that some developmental enhancers remain hypomethylated but become inactive in adult tissues [51] . It is still unclear whether DNA hypomethylation of enhancers are necessary for their activities or hypomethylation is a result of enhancer activation by another mechanism [14] . Further investigation will be required to elucidate the precise relationship between DNA methylation and enhancer activity. Collection of embryos and isolation of genomic DNA All zebrafish were used in accordance with the protocols approved by the Washington University Animal Studies Committee (Protocol 20110236). Wild-type sjA strain zebrafish were maintained under standard conditions [58] . Sperm were collected from sexually mature zebrafish males by standard protocol [58] . Wild-type embryos were obtained through in vitro fertilization, grown in 28.5 °C egg water (60 μg ml −1 Ocean Sea Salts) to develop to the desired stages and harvested at five different developmental stages: 256-cell (~2.5 hpf), 1K cell-High (~3.5 hpf), dome (~4.5 hpf), shield (~6 hpf) and 24 hpf. Chorions were removed with pronase and yolk was removed with ice-cold deyolking buffer (55 mM NaCl, 1.8 mM KCl, 1.25 mM NaHCO 3 ). Embryos were snap-frozen in liquid nitrogen and stored at −80 °C until the time of use. The genomic DNA was isolated by incubating embryos in genomic DNA extraction buffer (50 mM Tris, 1 mM EDTA, 0.5% SDS, 1 mg ml −1 Proteinase K) followed by phenol–chloroform extraction. DNA concentrations and purity were measured using NanoVue (GE Healthcare Life Sciences) and DNA integrity was confirmed by gel electrophoresis. MeDIP and MRE-seq library generation and sequencing MeDIP and MRE-seq libraries were generated as described previously [18] , [59] , with minor modifications. For MeDIP-seq, 500 ng of DNA isolated was sonicated to a fragment size of 100–500 bp, end processed and ligated to paired-end adapters. After agarose gel size selection of 166–566 bp, DNA was heat denatured and then immunoprecipitated using a mouse monoclonal anti-methylcytidine antibody (1 μg of antibody per 1 μg of DNA, Eurogentec) in 500 μl of immunoprecipitation buffer (10 μM sodium phosphate, pH 7.0, 140 mM sodium chloride and 0.05% Triton X-100) overnight at 4 °C. Antibody/DNA complexes were isolated by addition of 1 μl of rabbit anti-mouse IgG secondary antibody (2.4 mg ml −1 , Jackson Immunoresearch) and 100 μl protein A/G agarose beads (Pierce Biotechnology) for 2 h at 4 °C. Beads were washed six times with immunoprecipitation buffer and then DNA was eluted in TE buffer with 0.25% SDS and 0.25 mg ml −1 of proteinase K for 2 h at 50 °C. DNA was then purified with QIAquick purification kit (Qiagen) and eluted in 30 μl EB buffer. DNA was amplified by 12 cycles of PCR with the standard Illumina index primers and size selected (220–620 bp) by agarose gel electrophoresis. For MRE-seq, five parallel digests (HpaII, Hin6I, SsiI, BstUI and HpyCH4IV; New England Biolabs) were performed, each with 200 ng of DNA. Five units of enzyme were initially incubated with DNA for 3 h and then additional five units of enzyme were added to the digestion for a total of 6 h of digestion time. DNA was purified by phenol/chloroform/isoamyl alcohol extraction, followed by chloroform extraction using phase lock gels. Digested DNA from the different reactions was combined and precipitated with 1/10 volume of 3 M sodium acetate (pH 5.2) and 2.5 volumes of ethanol. The purified DNA was size selected (100–500 bp), end processed and ligated to single-end adapters. After the second size-selection procedure (166–566 bp), DNA was amplified by 15 cycles of PCR and size selected (220–620 bp) by agarose gel electrophoresis. MeDIP and MRE libraries were sequenced on Illumina HiSeq machine, with a total number of ~540 million MeDIP-seq reads and 300 million MRE-seq reads. These reads were mapped to the latest zebrafish genome assembly (Zv9) by using Novoalign (Novocraft). Estimation of methylation levels at single CpG resolution Methylation levels at single CpG resolution were estimated by using methylCRF with default parameters [33] , [59] . The methylCRF scores of 24,222,562 CpGs in 26 chromosomes were calculated and 1,028,605 CpGs in scaffolds were excluded. Concordance between MethylC-seq and methylCRF predictions was measured by calculating the differences of predictions on the same CpG sites from the matched samples. The CpGs whose methylation levels do not exist in MethylC-seq were excluded in concordance calculation. The average DNA methylation levels over different genic or genomic features were calculated per CpG in 30 bins per genic or genomic feature. Gene coordinates were obtained from zebrafish gene set of Ensembl release 71 and promoter was defined as 1 kb upstream region from the TSS. CGI annotation was obtained from the UCSC Genome Browser CGI track. CGI shores and CGI shelves were defined as regions 2 kb up and downstream of the CGIs and CGI shores, respectively. LncRNA gene annotations were obtained from the recent zebrafish lncRNA study [40] . To classify promoters in two categories, HCPs and LCPs, we first determined the GC content and the ratio of observed versus expected (o/e) CpG in sliding 500-bp windows with 5-bp offset for each 1 kb upstream TSS region. The o/e CpG ratio was calculated by the following formula: (number of CpGs times number of bp)/(number of Cs times number of Gs) [35] . The promoters were classified as HCPs if the promoters contain a subsequence with an o/e CpG ratio of ≥0.65 and a GC content of >0.30, and were classified as LCPs if they did not meet these criteria. More than half of the promoters were classified as HCPs ( Supplementary Fig. 8a ). The average DNA methylation levels over 4-kb regions around the TSS were calculated per CpG in 100-bp bins ( Supplementary Fig. 8b ). Targeted validation of the methylation levels Genomic DNA underwent bisulfite conversion using EpiTect Bisulfite Kit (Qiagen), following the manufacturer’s instructions. Regions of interest were amplified with specific PCR primers ( Supplementary Table 7 ), using HiFi HotStart Uracil+ ReadyMix (Kapa Biosystems). For clonal Sanger sequencing, amplified regions were cloned into pCR4-TOPO vector (Invitrogen) and more than 15 bacterial clones were used for Sanger sequencing. For pyrosequencing, amplified regions were subjected to pyrosequencing reaction in PyroMark Q24 (Qiagen) with specific sequencing primers ( Supplementary Table 7 ), following the manufacturer’s instructions. Data were analysed with the PyroMark Q24 software (Qiagen). Analysis of DMRs DMRs between developmental stages were identified by using methylMnM package [23] , [59] with the default parameters in R environment. Briefly, the coverage of MeDIP and MRE sequencing data and genomic CpG information were calculated in each 500-bp genomic bin. Scaffolds and the mitochondrial genome were excluded from the analysis. DMRs with a Q -value <1 × 10 −5 were selected for analysis. The complete list of dsDMRs are accessible at http://epigenome.wustl.edu/Zebrafish_DNAme/ . The average methylation level of CpGs in each DMR was calculated using methylCRF scores and the differences of methylation scores between two developmental stages were calculated. To annotate dsDMRs, we first divided the zebrafish genome into the four non-overlapping genomic features based on the following criteria. Gene annotation was obtained from zebrafish gene set of Ensembl release 71. The longest transcript was chosen from multiple transcripts for each protein-coding gene. Promoters were defined as 1.5 kb upstream and 0.5 kb downstream region from TSS of each protein-coding gene. Exons and introns were defined as annotated in Ensembl release 71, excluding regions that were defined as promoters. All the remaining genomic regions were defined as intergenic. Each dsDMR was annotated as one of the four genomic features if the centre of the dsDMR resides within the corresponding genomic feature. To investigate the distribution of dsDMRs around developmental genes, we first chose the 772 genes under the GO term ‘GO0009790: embryo development’. We also randomly chose the same number of protein-coding genes. We calculated the number of dsDMRs in a 10-kb window upstream of the TSS of each gene selected. We then calculated the mean number of dsDMRs for each 10-kb windows over the 772 genes and generated the average dsDMR distribution plot. For evolutionary conservation analysis, the vertebrate PhastCons score based on the eight-way vertebrate genome alignment was obtained from the UCSC Genome Browser PhastCons conservation track. Histone modification ChIP-seq data were obtained from the recent study [38] . Analysis of dsDMRs as developmental enhancers GO enrichment was performed using the GREAT analysis tool [39] . Gene regulatory domains were defined by default as the following: basal regulatory domain was defined as a region spanning 5 kb upstream of and 1 kb downstream from the TSS; the distal regulatory domain was then extended in both directions to the nearest gene’s basal domain but not more than 1,000 kb in one direction. The GO terms that have a minimum of 2.5-fold region-based enrichment and that have a false discovery rate below 0.05 were reported. For gene expression analysis, the RNA-seq data were obtained from a recent study [40] . The RNA-seq reads were mapped to the zebrafish genome assembly Zv9 by using tophat [60] and FPKM values were calculated for each gene by using cufflinks [61] . TF-binding motif enrichment analysis Motif enrichment analysis in dsDMRs was performed using the HOMER tool [62] . HOMER scanned the sequences of dsDMRs for known motifs, including HOMER-provided motifs library and JASPAR core vertebrate motifs [63] , and calculated enrichment score P -values using hypergeometric test. DAVID tool [64] was used to functionally annotate the TFs whose motifs are enriched in dsDMRs. The zebrafish Ensemble gene IDs corresponding to the enriched motifs were used as input for DAVID tool. The entire zebrafish genome was first used as background for DAVID. As many GO terms related to transcription activities were enriched against this background ( Supplementary Fig. 14 ), all TFs from motif enrichment analysis were also used as background for DAVID ( Supplementary Fig. 15a ). Construction of gene regulatory network To obtain the regulatory interactions among the putative target genes and TFs identified from dsDMRs, these genes and TFs were used as nodes in the UCSC Interaction Browser [65] as described previously [66] , with minor modifications as detailed below. First, 215 genes were identified as putative targets of dsDMR enhancers by their association with dsDMRs from GREAT analysis. Next, 49 TFs whose motifs were enriched in dsDMRs were included as additional nodes. Two network collection databases were used to query for interactions among the genes: GEA_CLR network connecting TF to targets [67] and ChEA TF network [68] . To compute statistical significance, 10 sets of 215 random genes and 49 random TFs were used as nodes and an expected distribution of connections among the given number of genes was obtained (mean of 1,886 and s.d. of 260; Supplementary Fig. 15b ). To build putative regulatory network of the eye development, TFs were first linked to the target genes. TFs related with the eye development were selected from the TFs with enriched motifs. Target genes related with the eye development were selected from the gene list identified from GREAT analysis. A TF whose motif is in a dsDMR was linked to a gene to which GREAT associate the dsDMR. The known target genes of sox2 were from the ChEA system [68] . Zebrafish in vivo enhancer assay Putative enhancer sequences were PCR amplified with specific primers ( Supplementary Table 3 ) and TOPO-cloned into an entry vector (pCR8/GW/TOPO, Invitrogen) of the Gateway cloning system. The cloned plasmid was then recombined with the destination vector (pGW_cfosEGFP, generous gift from Shannon Fisher) to generate the desired reporter plasmid. Prepared plasmid DNAs for microinjection were further purified with QIAquick spin columns (Qiagen). Tol2 transposase mRNA was transcribed in vitro from the pCS-Tp vector [46] (a generous gift from Shannon Fisher), using the mMessage mMachine Sp6 kit (Ambion). Embryos at one-cell or two-cell stages were injected with transposase mRNA, transposon plasmid DNA and phenol red solution as described previously [45] . At least 100 embryos were injected for each construct. The reporter expression patterns were analysed at 24 hpf stage. If >10% of embryos exhibit the consistent GFP expression pattern, the construct was considered as a positive enhancer. The embryos with specific expression patterns were selected and raised to sexual maturity. Sexually mature G0 adults were crossed with sjA wild-type strain to obtain germline transmission. Two or more independent G1 transgenic lines were established for each construct, unless otherwise indicated. G1 transgenic fish embryos were photographed at 24 hpf stage. Accession codes: The MeDIP-seq and MRE-seq data from this study have been deposited to the NCBI Gene Expression Omnibus (GEO) under accession number GSE52706 , containing the Subseries GSE52703 (MeDIP-seq) and GSE52704 (MRE-seq). How to cite this article: Lee, H. J. et al. Developmental enhancers revealed by extensive DNA methylome maps of zebrafish early embryos. Nat. Commun. 6:6315 doi: 10.1038/ncomms7315 (2015).